Correlated defect nanoregions in a metal–organic framework Throughout much of condensed matter science, correlated disorder is a key to material function. While structural and compositional defects are known to exist within a variety of metal–organic frameworks (MOFs), the prevailing understanding is that these defects are only ever included in a random manner. Here we show—using a combination of diffuse scattering, electron microscopy, anomalous X-ray scattering and pair distribution function measurements—that correlations between defects can in fact be introduced and controlled within a hafnium terephthalate MOF. The nanoscale defect structures that emerge are an analogue of correlated Schottky vacancies in rocksalt-structured transition metal monoxides and have implications for storage, transport, optical and mechanical responses. Our results suggest how the diffraction behaviour of some MOFs might be reinterpreted, and establish a strategy of exploiting correlated nanoscale disorder as a targetable and desirable motif in MOF design. The incorporation of point defects within an ordered material gives rise to local fields (for example, strain, electrostatic, dipolar, chemical potential) that form the basis of a wide range of useful functionalities; examples include the polar nanoregions of relaxor ferroelectrics [1] , collective orbital fluctuations in the colossal magnetoresistive manganites [2] , and cooperative charge transport mechanisms in superionic conductors [3] . While even non-interacting defects can affect bulk material properties such as density and/or porosity, arguably the most interesting phenomena emerge from collective states where local fields associated with individual defects interact with one another. The control of semiconductor electron transport properties by judicious electron/hole doping is one example; low-barrier cooperative oxide–conduction pathways in fuel cell materials another [4] ; doping-driven stabilization of relaxor behaviour in ferroelectrics a third [1] . Whether or not defect interactions are expected to occur depends on two principal factors: defect concentration, and the effective size of the corresponding defect field. As part of the concerted research effort into developing new classes of functional materials that exploit the diverse nature of metal–organic framework (MOF) chemistry, it has now emerged that structural and compositional defects can be included within a variety of MOF families [5] , [6] , [7] , [8] , [9] . If correlated defect structures are ever to be exploited in designing functional MOFs, it remains to be shown that sufficiently high defect concentrations and field strengths can be attained in these systems. The few existing studies of defective MOFs have so far employed either one of two different approaches: ligand–fragment coassembly to increase pore accessible volume and adsorption site density on the one hand [5] , [6] , and mesoscale texturing via surfactant inclusion [7] , [10] on the other hand. In neither case have defect correlations yet been observed. It was in this context that the recent report of substantial (~\n10%) non-stoichiometry in the zirconium MOF UiO-66 piqued our interest [11] , [12] . This material—favoured among MOFs for its attractive thermal, mechanical and chemical stability [13] , [14] —has the nominal chemical formula [Zr 6 O 4 (OH) 4 ][C 6 H 4 (COO) 2 ] 6 s˙{guest}. In its crystal structure, six-centred zirconium oxyhydroxide clusters are linked via terephthalate (1,4-benzenedicarboxylate) bridges to form a face-centred-cubic ( fcu ) net ( Fig. 1 ). This net is notable [15] for its high degree of topological connectivity (12 connected nodes), a design feature considered responsible for the unusually high thermal and chemical stability of this system [13] . Like many other canonical MOFs, UiO-66 forms the basis of an isoreticular family: Hf or U can substitute Zr [16] , [17] , and a number of different dicarboxylates can be used in lieu of the terephthalate anion [13] , [18] . The first indication of non-stoichiometry came from thermogravimetric analysis (TGA) measurements, which suggested that approximately one in 12 of the terephthalate linkers supposedly bound to each [Zr 6 O 4 (OH) 4 ] cluster was in fact missing [11] . A subsequent high-resolution neutron scattering study, in which relative site occupancies were determined, supported precisely this same interpretation [12] . Moreover, by varying during synthesis the concentration of monocarboxylic acid ‘modulators’—usually considered to play only the ‘spectator’ role of ameliorating crystallization kinetics [19] —it has now been shown that vacancy concentrations can be controlled in a systematic manner [12] , [20] . 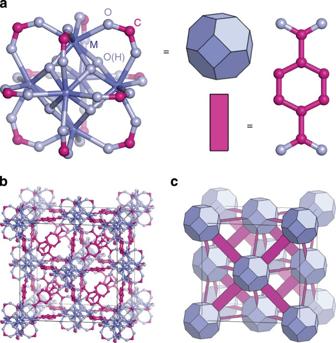Figure 1:Structural description of UiO-66MOFs. (a) The fundamental building unit of the UiO-66 framework type is a six-centre octahedral metal cluster, in which eight-coordinate cations (M) are connected via carboxylate linkers. Capping the faces of each M6octahedron are eight μ3-O bridges, of which four are protonated to account for charge balance. M atoms are shown in dark blue, O atoms in light blue and C atoms in magenta. Terephthalate (1,4-benzenedicarboxylate) linkers (a, right) connect these units such that the clusters adopt an expanded face-centred-cubic arrangement, as shown inb. In thisfcutopology, each cluster is connected to 12 neighbouring clusters by terephthalate linkers. The colour scheme is as ina; hydrogen atoms are omitted for clarity. (c) A simplified polyhedral representation of the same network structure. The blue truncated octahedra and magenta rectangles correspond, respectively, to M6cluster coordination polyhedra and terephthalate linkers. Figure 1: Structural description of UiO-66 MOFs. ( a ) The fundamental building unit of the UiO-66 framework type is a six-centre octahedral metal cluster, in which eight-coordinate cations (M) are connected via carboxylate linkers. Capping the faces of each M 6 octahedron are eight μ 3 -O bridges, of which four are protonated to account for charge balance. M atoms are shown in dark blue, O atoms in light blue and C atoms in magenta. Terephthalate (1,4-benzenedicarboxylate) linkers ( a , right) connect these units such that the clusters adopt an expanded face-centred-cubic arrangement, as shown in b . In this fcu topology, each cluster is connected to 12 neighbouring clusters by terephthalate linkers. The colour scheme is as in a ; hydrogen atoms are omitted for clarity. ( c ) A simplified polyhedral representation of the same network structure. The blue truncated octahedra and magenta rectangles correspond, respectively, to M 6 cluster coordination polyhedra and terephthalate linkers. Full size image That correlations between vacancy defects might play an important role in this family was suggested to us by the appearance of structured diffuse scattering in the powder diffraction profile of UiO-66(Hf) [16] . This diffuse scattering takes the form of weak, broad, superlattice peaks centred on scattering positions associated with primitive ( hkl ) reflections that are forbidden for the face-centred-cubic structure of the parent framework. In the study of ref. 16 , these diffuse scattering peaks are attributed to the presence of disordered solvent and consequently were not accounted for in the accompanying structural analysis. The analysis of structured diffuse scattering—particularly in powder diffraction patterns—is notoriously difficult: by its very nature, the scattering arises from structural motifs that have only short-range correlations, and so conventional crystallographic approaches (which rely on long-range periodicity) are not generally applicable [21] . The increasing availability of methods for modelling nanoscale disorder within the crystalline materials does, however, allow some considerable progress to be made [22] , [23] . Conventionally (when studying disorder in oxide frameworks, for example), high-resolution electron microscopy methods might be used to probe the periodicity and reflection conditions associated with diffuse scattering [24] , and in especially favourable cases may even allow resolution of individual defects in real space [25] ; likewise, for systems available as sufficiently large single crystals, single-crystal X-ray diffraction measurements can also provide extremely valuable insight into the defect structures responsible for the diffuse scattering observed [26] . Unfortunately, neither technique is straightforwardly applicable to studying UiO-66(Hf) given the susceptibility of MOFs to damage in the electron beam and also the unavailability of single-crystal samples. Yet, the key point remains: namely, that the diffuse scattering contribution to the diffraction pattern contains useful and analyzable information concerning the particular short-range structural order from which it arises [24] . In this study, we apply a range of experimental and computational techniques to the problem of understanding correlated disorder in UiO-66(Hf). We show that the diffuse scattering observed experimentally cannot be understood completely in terms of solvent inclusion and/or linker vacancies but arises instead from correlated vacancies of Hf 6 clusters. By varying the relative concentrations of modulator and linker components, we observe systematic changes in both the coherence length and volume fraction of defect nanoregions. In this way, we demonstrate not only that correlated defect structures indeed occur within this metal–MOF, but also that the particular form of that defect structure can be controlled synthetically. Superlattice reflections We prepared a sample of polycrystalline UiO-66(Hf) using the approach outlined in refs 11 , 12 , 16 , 20 where we also included a large excess of formic acid modulator to encourage defect formation. X-ray powder diffraction measurements of our product gave a diffraction pattern that was essentially identical to that reported in ref. 16 ( Fig. 2a ); in particular, we also observed the coexistence of sharp Bragg peaks for all parent ( hkl ) reflections ( h + k , k + l and h + l =2 n ) and weak, broad, diffuse features for primitive superlattice peaks ( h + k , k + l or h + l =2 n +1). By varying the relative concentrations of formic acid modulator and terephthalate linker, we were able to access UiO-66(Hf) products that gave diffraction patterns with essentially the same parent Bragg intensities, but with different relative intensities of the diffuse component ( Fig. 2 ). This variation in relative intensities was in fact systematic: the diffuse component is always most noticeable for high formic acid and/or low terephthalate compositions ( Fig. 2f,g ). We can rule out the possibility that our product (and presumably that of ref. 16 ) consists of two phases—namely, a crystalline, face-centred-cubic UiO-66 phase and a second, nanocrystalline, primitive cubic variant of the UiO-66 structure—on the basis of its behaviour in the electron microscope. While our samples are too beam-sensitive to survive investigation using high-resolution transmission electron microscopy, the electron diffraction patterns of individual UiO-66(Hf) crystallites could be taken and were found to include both parent and superlattice reflections ( Fig. 3a,b , Supplementary Figs 1–4 ). Anomalous X-ray scattering measurements offer further insight into the chemical origin of these superlattice reflections: comparison of X-ray powder diffraction patterns measured away from and on the Hf K-absorption edge reveals a subtle but reproducible variation in the superlattice reflection intensities ( Fig. 3c,d ) that is consistent with a modulation in the occupancy of Hf sites but that would not be expected were the diffuse scattering to arise from solvent ordering and/or linker vacancies alone ( Supplementary Fig. 5 , Supplementary Discussion ). X-ray pair distribution function (PDF) measurements suggest there is no significant change in the local structure of the Hf-containing clusters between defective and defect-free UiO-66(Hf) samples ( Fig. 3e ); consequently, any modulation in Hf occupancy within the defective samples would appear to involve variation in the concentration of entire cluster units. Taken together, the above observations suggest (i) the diffuse scattering arises (at least partially) from variations in the scattering contribution of Hf 6 oxyhydroxide clusters, (ii) there exists a short-range-ordered structural modification to the hafnium terephthalate framework with a periodicity characterized by the primitive lattice vectors (1,0,0)*, and (iii) that the extent of this modification depends on the relative concentration of formate modulator and terephthalate linker used during framework synthesis. So, just as the authors of ref. 12 found modulator concentration to affect vacancy concentration, here we find it to control the extent of short-range structural correlations. 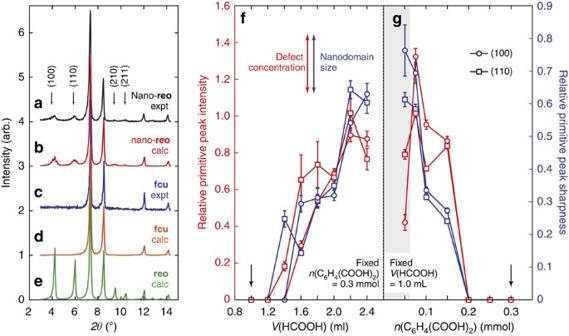Figure 2: Chemical control over defect nanoregion concentration and domain size. (a) The experimental low-angle X-ray diffraction pattern of UiO-66(Hf), measured over the angular range 3–15° (λ=1.541 Å), consists of a sharp Bragg scattering component with reflections obeying the conditions expected for the face-centred-cubic lattice illustrated inFig. 1and a less-intense diffuse scattering component centred on ‘forbidden’ reflection positions associated with a primitive cubic superstructure. The four most intense diffuse scattering peaks are highlighted by arrows. Conventional crystallographic analysis of this pattern is illustrated inSupplementary Fig. 29. (b) The corresponding diffraction pattern calculated from thereodefect nanoregion model described in the text: the intensities and peak widths of both Bragg and diffuse scattering contributions are quantitatively accounted for by this model. The experimental (c) and calculated (d) diffraction patterns for a defect-freefcuframework, showing the absence of diffuse scattering features. (e) A long-range-orderedreomodel gives rise to superlattice peaks in the same positions as those observed ina, but simultaneously overestimates peak intensities and underestimates peak widths. Instead, the relative intensities and widths of the diffuse superlattice reflections measure defect concentration and domain size, respectively. (f) Increasing modulator (formic acid) concentration for fixed linker concentration during synthesis results in a higher concentration ofreonanoregions of increasing domain size, as does (g) decreasing linker concentration for fixed modulator concentration. Points of identical composition are indicated by arrows; the shaded region ingcorresponds to compositions for which additional phases are present. For all data points ingandh, the solvothermal reaction conditions used were as follows: 48 h, 120 °C, 4 ml DMF, 0.3 mmol HfCl4; HCOOH and C6H4(COOH)2concentrations as indicated in the plots. Relative primitive peak sharpness values (blue data points) were determined as the ratio of peak widthsσ(111)/σ(100) andσ(111)/σ(110) extracted from Pawley profile fitting; relative primitive peak intensities (red data points) were determined as the ratio of observed primitive peak intensity to the extrapolated value at maximum defect concentration. The error bars represent standard uncertainties in the mean values. Figure 2: Chemical control over defect nanoregion concentration and domain size. ( a ) The experimental low-angle X-ray diffraction pattern of UiO-66(Hf), measured over the angular range 3–15° ( λ =1.541 Å), consists of a sharp Bragg scattering component with reflections obeying the conditions expected for the face-centred-cubic lattice illustrated in Fig. 1 and a less-intense diffuse scattering component centred on ‘forbidden’ reflection positions associated with a primitive cubic superstructure. The four most intense diffuse scattering peaks are highlighted by arrows. Conventional crystallographic analysis of this pattern is illustrated in Supplementary Fig. 29 . ( b ) The corresponding diffraction pattern calculated from the reo defect nanoregion model described in the text: the intensities and peak widths of both Bragg and diffuse scattering contributions are quantitatively accounted for by this model. The experimental ( c ) and calculated ( d ) diffraction patterns for a defect-free fcu framework, showing the absence of diffuse scattering features. ( e ) A long-range-ordered reo model gives rise to superlattice peaks in the same positions as those observed in a , but simultaneously overestimates peak intensities and underestimates peak widths. Instead, the relative intensities and widths of the diffuse superlattice reflections measure defect concentration and domain size, respectively. ( f ) Increasing modulator (formic acid) concentration for fixed linker concentration during synthesis results in a higher concentration of reo nanoregions of increasing domain size, as does ( g ) decreasing linker concentration for fixed modulator concentration. Points of identical composition are indicated by arrows; the shaded region in g corresponds to compositions for which additional phases are present. For all data points in g and h , the solvothermal reaction conditions used were as follows: 48 h, 120 °C, 4 ml DMF, 0.3 mmol HfCl 4 ; HCOOH and C 6 H 4 (COOH) 2 concentrations as indicated in the plots. Relative primitive peak sharpness values (blue data points) were determined as the ratio of peak widths σ (111)/ σ (100) and σ (111)/ σ (110) extracted from Pawley profile fitting; relative primitive peak intensities (red data points) were determined as the ratio of observed primitive peak intensity to the extrapolated value at maximum defect concentration. The error bars represent standard uncertainties in the mean values. 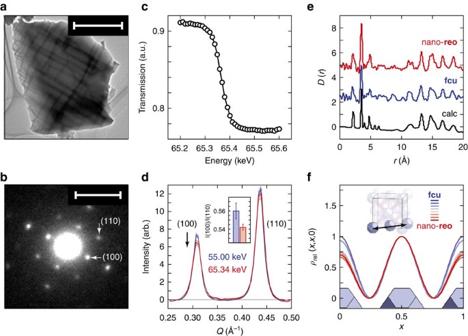Figure 3: Experimental characterization of correlated defect inclusion. (a) UiO-66(Hf) crystallites show a complex microstructure (domain sizeca0.1–0.4 μm) with domain walls oriented perpendicular to the (100) crystal axes; scale bar, 1 μm. The dark lines at domain boundaries correspond to planes of mass contrast viewed in cross-section and are too thin to contribute to the diffraction pattern (Supplementary Fig. 1a). (b) The selected area electron diffraction pattern of the same crystallite shows that the primitive superlattice peaks identified inFig. 2(i) do not arise from a separate phase and (ii) retain cubic symmetry; scale bar, 0.1 Å−1(1/d; that isQ=0.63 Å−1). The particular example shown here is for the sample with largest defect concentration and nanodomain size. Note that any diffraction texture arising from the microstructure in (a) corresponds to periodicities of the order of 10−3Å−1, which is small with respect to the scale used in (b) and the diffraction patterns reported inFig. 2. (c) Location of the X-ray absorption edge associated with the Hf K transition, determined using transmission measurements of the nano-reoUiO-66(Hf) phase. (d) Anomalous X-ray scattering at the Hf K-edge (65.34 keV) results in a small (1–5%) variation in background-subtracted diffraction intensities relative to off-edge measurements (here, 55 keV) for those peaks to which Hf scattering contributes, seen here to include the superlattice reflections. The inset shows the difference in the ratioI(100)/I(110) at these two energies. (e) As a result of the large Hf X-ray scattering cross-section, X-ray PDF measurements are dominated by Hf pair correlations; these correlations show the local Hf coordination environment (that is, cluster geometry) is similar in nano-reo(top, raised by 5 units) and non-defectivefcu(middle, raised by 2.5 units) UiO-66(Hf) samples, and is well-modelled by the structure determined crystallographically (bottom). (f) Coarse-grained Fourier maps reconstructed from the low-angle diffraction patterns ofFig. 2reveal a systematic decrease in scattering intensity at the unit cell origin with increasing defect concentration that is consistent with short-range ordering of cluster vacancies on the primitive cubic lattice. Full size image Figure 3: Experimental characterization of correlated defect inclusion. ( a ) UiO-66(Hf) crystallites show a complex microstructure (domain size ca 0.1–0.4 μm) with domain walls oriented perpendicular to the (100) crystal axes; scale bar, 1 μm. The dark lines at domain boundaries correspond to planes of mass contrast viewed in cross-section and are too thin to contribute to the diffraction pattern ( Supplementary Fig. 1a ). ( b ) The selected area electron diffraction pattern of the same crystallite shows that the primitive superlattice peaks identified in Fig. 2 (i) do not arise from a separate phase and (ii) retain cubic symmetry; scale bar, 0.1 Å −1 (1/ d ; that is Q =0.63 Å −1 ). The particular example shown here is for the sample with largest defect concentration and nanodomain size. Note that any diffraction texture arising from the microstructure in ( a ) corresponds to periodicities of the order of 10 −3 Å −1 , which is small with respect to the scale used in ( b ) and the diffraction patterns reported in Fig. 2 . ( c ) Location of the X-ray absorption edge associated with the Hf K transition, determined using transmission measurements of the nano- reo UiO-66(Hf) phase. ( d ) Anomalous X-ray scattering at the Hf K-edge (65.34 keV) results in a small (1–5%) variation in background-subtracted diffraction intensities relative to off-edge measurements (here, 55 keV) for those peaks to which Hf scattering contributes, seen here to include the superlattice reflections. The inset shows the difference in the ratio I (100)/ I (110) at these two energies. ( e ) As a result of the large Hf X-ray scattering cross-section, X-ray PDF measurements are dominated by Hf pair correlations; these correlations show the local Hf coordination environment (that is, cluster geometry) is similar in nano- reo (top, raised by 5 units) and non-defective fcu (middle, raised by 2.5 units) UiO-66(Hf) samples, and is well-modelled by the structure determined crystallographically (bottom). ( f ) Coarse-grained Fourier maps reconstructed from the low-angle diffraction patterns of Fig. 2 reveal a systematic decrease in scattering intensity at the unit cell origin with increasing defect concentration that is consistent with short-range ordering of cluster vacancies on the primitive cubic lattice. Full size image Structural description of defect nanoregions The question remains: what exactly are the short-range correlations responsible for the diffuse scattering we observe? Just as systematic absences in the Bragg diffraction patterns of long-range-ordered materials place strong constraints on the corresponding real-space structures, so too does the form of diffuse scattering we observe allow us to draw conclusions regarding the short-range correlations present in our UiO-66(Hf) samples. A picture in which linker vacancies of the type suggested in refs 11 , 12 , 20 are correlated with appropriate periodicity is an attractive model to explain the diffuse scattering, but is inconsistent with our anomalous X-ray scattering measurements; moreover, local structure refinements that allow vacancies only on the linker sites cannot account for the existence of scattering intensity at the (110) position or indeed any reflection satisfying h + k + l =2 n ( Supplementary Fig. 5 ). Vacancies at the cluster sites themselves, however, would be consistent with both the anomalous scattering and the diffuse reflection conditions. It can be shown that there are only two possible cluster vacancy modifications to the face-centred-cubic structure that are characterized by (1,0,0)* periodicities and that preserve cubic symmetry (the electron diffraction patterns indicating that this is retained): one is the ordering of vacancies on the face-centred sites, leaving unconnected Hf 6 clusters only at the corners of the unit cell; the other is the inverse situation where vacancies order at the corners of the cubic unit cell to give a locally eight-connected net with reo topology ( Fig. 4a ). The former is clearly unphysical, because it would require isolated clusters to remain spatially correlated across nanometre-scale voids, whereas a long-range-ordered version of the latter is actually known to occur in the related DUT-51(Zr) framework [27] . Furthermore, coarse-grained Fourier maps reconstructed from the low-angle diffraction intensities of Fig. 2 also suggest decreasing cluster occupation at the unit cell origin relative to the face-centred sites with increasing defect concentration ( Fig. 3f , Supplementary Fig. 6 ). Consequently, we sought to determine whether a short-range (nano-correlated) reo model can actually account quantitatively for the diffuse scattering features observed. In developing such a model, there are only two parameters to be determined—the fraction of cluster vacancies and the reo domain size. These are in turn constrained by the relative intensities and widths of the four principal diffuse scattering peaks (that is, eight measurable quantities). Comparison of observed and calculated diffuse peak widths and intensities allows us to estimate an effective vacancy fraction and reo domain size for our original UiO-66(Hf) sample of 0.13(5) and 7(3) nm, respectively ( Supplementary Methods , Supplementary Fig. 7 ). From these parameters, we can construct an atomistic model that accounts successfully for both the sharp Bragg peaks and the broad diffuse scattering component in the powder diffraction pattern ( Figs 2b , 4 ). 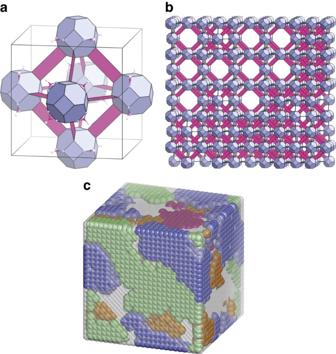Figure 4: Structural description of defect nanoregions in UiO-66(Hf). (a) A polyhedral representation of a single-unit cell of the (ordered)reodefect structure, using the same colour scheme employed inFig. 1cand making use of the atomic coordinates and unit cell parameters extracted from the equilibrium structure obtained in our density functional theory calculations (Supplementary Table 10). In this model, 25% of the cluster sites are vacant and the cluster coordination number is reduced from 12 to 8. The clusters occupy Nb sites in the defect-vacancy structure of the transition metal monoxide NbO. (b) A representative section of the atomistic model from which the simulated diffraction pattern shown inFig. 2bis generated. Defect-rich nanoregions are dispersed throughout a matrix of defect-freefcuframework. (c) The defect concentration and domain size parameters determined experimentally can be used to generate atomistic representations of defect nanoregions in UiO-66(Hf). The representation given here is for a 6 × 6 × 6 supercell of thefcuunit cell (total edge length 12.4 nm), chosen for clarity to be smaller by a factor of 43than those configurations used to calculate the diffraction pattern shown inFig. 2b. There are four possible orientations of thereodefect structure relative to the bulkfcuframework, corresponding to the four cluster positions in thefcuunit cell. In the representation used here, individual clusters are not shown but nanodomains corresponding to each of these four orientations are represented by blue, green, orange and magenta regions. Grey-coloured regions correspond to defect-freefcuframework. Figure 4: Structural description of defect nanoregions in UiO-66(Hf). ( a ) A polyhedral representation of a single-unit cell of the (ordered) reo defect structure, using the same colour scheme employed in Fig. 1c and making use of the atomic coordinates and unit cell parameters extracted from the equilibrium structure obtained in our density functional theory calculations ( Supplementary Table 10 ). In this model, 25% of the cluster sites are vacant and the cluster coordination number is reduced from 12 to 8. The clusters occupy Nb sites in the defect-vacancy structure of the transition metal monoxide NbO. ( b ) A representative section of the atomistic model from which the simulated diffraction pattern shown in Fig. 2b is generated. Defect-rich nanoregions are dispersed throughout a matrix of defect-free fcu framework. ( c ) The defect concentration and domain size parameters determined experimentally can be used to generate atomistic representations of defect nanoregions in UiO-66(Hf). The representation given here is for a 6 × 6 × 6 supercell of the fcu unit cell (total edge length 12.4 nm), chosen for clarity to be smaller by a factor of 4 3 than those configurations used to calculate the diffraction pattern shown in Fig. 2b . There are four possible orientations of the reo defect structure relative to the bulk fcu framework, corresponding to the four cluster positions in the fcu unit cell. In the representation used here, individual clusters are not shown but nanodomains corresponding to each of these four orientations are represented by blue, green, orange and magenta regions. Grey-coloured regions correspond to defect-free fcu framework. Full size image Defect formation and quantum mechanical calculations Inspection of the model ( Fig. 4 ) helps us understand the microscopic mechanism responsible for ordered vacancy inclusion. First, the superlattice reflection intensities suggest ~\n50% of the Hf 6 clusters are located within or adjacent to reo -type nanoregions, with individual domains dispersed throughout a continuous 12-coordinate fcu network ( Supplementary Methods ). There are four equally populated domain orientations corresponding to the four lattice sites in the face-centred-cubic cell ( Fig. 4c ). Within each reo domain, the Hf 6 clusters are coordinated by not fewer than eight terephthalate linkers (noting that additional linker vacancies may reduce this number further). The sensitivity of X-ray diffraction intensities to the nature of the species bound at the remaining coordination sites is very low, but from a chemical viewpoint one expects these sites to be occupied by formate anions. The tendency to adopt a lower effective cluster coordination number in the presence of increased formate concentration will be driven largely by a shift in the equilibrium position of the reaction equation but will perhaps also be encouraged by steric and statistical considerations. The balance between different ordered and nanoscale reo / fcu structures suggests the kinetics of domain nucleation, growth and ligand diffusion may well play a role in determining product composition. Exploring this possibility further, we find experimentally that, by extending the reaction time for a given reaction mixture, the defect nanoregions grow in size, increasing the observed correlation length ( Supplementary Fig. 8 ). This observation likely explains why diffuse primitive reflections have sometimes been observed and other times not been observed in previous experimental investigations [13] . So, in the presence of a suitable modulator concentration, UiO-66(Hf) growth appears to involve kinetically favoured formation of low-coordinate reo -type nanodomains that agglomerate into larger pseudocrystalline monoliths. Despite the lack of exact structural registration between individual nanodomain orientations, the lattice symmetry is such that X-ray diffraction patterns will still contain sharp Bragg reflections at d -spacings associated with the parent face-centred lattice; it is only the set of broad ‘reflections’ at disallowed (primitive) d -spacings that is sensitive to the concentration and coherence length of the individual reo nanodomains. The apparent miscibility of reo and fcu components is explained by density functional theory calculations: not only do we find the reo defect structure to be stable, but its unit cell dimensions differ from those of the parent fcu structure by less than 0.05% ( Supplementary Table 1 ). The model we have developed here differs from previous interpretations of disorder in the UiO family in two important respects. The first—and most crucial—is that we have shown that vacancy inclusion in UiO-66(Hf) proceeds in a correlated matter: the position of one vacancy affects the likelihood of vacancy inclusion at neighbouring sites. This demonstrates for the first time the possibility of designing MOFs that support correlated disordered states, such as are currently exploited in charge transport, catalysis, mechanical and optical responses of other longer-established solid-state materials families. Moreover, we have shown how these correlated states might be controlled from a synthetic viewpoint, and have explored their microscopic origin. The second difference is that we find vacancies at both the metal cluster and the linker sites—the entire network is more defective than had previously been imagined. This explains many of the apparent difficulties in interpreting gas sorption and TGA data ( Supplementary Figs 9–11 ) [12] . Of course, the key difficulty associated with estimating defect concentrations from Bragg intensities alone is that the total (node+linker) occupancy correlates with the overall scale factor; by contrast the relative intensities of diffuse and Bragg scattering are much more strongly sensitive to defect concentrations ( Supplementary Methods , Supplementary Fig. 5 ). So the vacancy model presented elsewhere on the basis of Rietveld refinement of neutron scattering intensities [12] , in which 11% of linker sites are deemed vacant, is actually indistinguishable on the basis of Bragg intensities from the reo -type cluster vacancy model with 33% occupancy (that is, 8% cluster vacancies). In fact, this ‘correlated defect nanoregion’ model we have determined for UiO-66(Hf) may be considered a MOF analogue of the Schottky defect phases of the transition metal monoxides [28] . For early transition metal monoxides, the most common defect structure adopted is the primitive NbO-type vacancy ordering, which produces both a structure and a diffraction pattern analogous to what we observe here for UiO-66(Hf) [28] . In the case of the monoxides, local defect ordering plays a crucial role in maximizing electronic conductivity [29] ; one anticipates the possibility of qualitatively similar effects on the band structure [12] and stabilities of UiO-66-type frameworks. Indeed our ab initio calculations also suggest a substantially reduced mechanical stiffness of the defective phase that will likely favour anomalous mechanical properties such as pressure-induced amorphisation and negative thermal expansion ( Supplementary Tables 2,3 ) [30] . A further consequence of the defect structure we observe is that it also introduces domain walls into the material on the nanometre scale. These features are likely to represent high-energy internal ‘surfaces’ with a propensity for increased chemical reactivity. The existence of such chemically active internal surfaces would be consistent with the solid-state ligand exchange found to occur under mild conditions in a number of materials within the broader UiO-66 family [31] . Finally, we note that the electron microscopy ( Fig. 3a ) indicates the existence of a complex microstructure within defective UiO-66(Hf) crystallites that concerns length scales not probed directly in the diffraction experiments we have performed but which may affect bulk material properties nonetheless, including sorption, transport and catalytic behaviour ( Supplementary Discussion , Supplementary Figs 12–15 ). It is improbable that UiO-66(Hf) is the only MOF to contain correlated defect nanoregions; rather, the relative difficulty of interpreting diffuse scattering patterns may have prevented more routine characterization of nanoscale structural complexity in a variety of MOF phases [32] . Yet there are a number of important consequences of correlated disorder in MOFs that we hope will motivate further study in this emerging field: mass transport pathways—and hence sorption profiles—might be affected by vacancy percolation; anomalous mechanical properties, such as negative thermal expansion, pressure-induced softening and crystalline–amorphous switching, are all more likely as correlated vacancies reduce network rigidity; electronic, magnetic, and optical functionalities are often favoured by engineering a delicate balance between charge ordered and disordered states; and, finally, the long-term goal of realizing complex active sites within MOFs for targeted catalysis relies explicitly on the ability to prearrange coordinatively unsaturated binding sites in a cooperative manner [9] . In all cases, nanoscale control over defect correlations promises the local structural and chemical complexity from which function ultimately arises. Sample preparation All reagents were obtained from commercial suppliers and used as supplied. Microcrystalline powders of UiO-66(Hf) were prepared using a solvothermal approach. Standard conditions for synthesis were as follows: HfCl 4 (0.3 mmol, 96 mg) and terephthalic acid (BDC; 0.3 mmol, 50 mg) were added to a PTFE-lined Parr reaction vessel (23 ml capacity), followed by N,N -dimethylformamide (DMF; 4 ml) and formic acid (95%, 1 ml). The vessel was sealed, heated at 120 °C for 48 h, then removed from the oven and allowed to cool to room temperature. The reaction mixture was subsequently filtered under vacuum and washed (acetone) to yield UiO-66(Hf) as a white microcrystalline powder. The stability of the sample and defect ordering to heat, solvent exchange, acid, base and attempted post-synthetic modification was also demonstrated (see Supplementary Figs 16–20 ). For the concentration studies shown in Fig. 2f,g , we adopted this basic procedure, modified as described below. Formic acid concentration study The quantity of formic acid was systematically varied from 1 to 2.4 ml in order to obtain the series of compounds on which the Fig. 2f is based, with each concentration point repeated in duplicate. As a consequence the total reaction mixture volume (solvent+formic acid) varied across the series. BDC, 0.3 mmol; formic acid, 1.0–2.4 ml; HfCl 4 , 0.3 mmol; DMF, 4 ml. BDC concentration study In a similar way, the quantity of BDC was systematically varied from 0.05 mmol to 0.3 mmol to obtain the series of compounds on which Fig. 2g is based. Again, all preparations were performed in duplicate. BDC, 0.05–0.3 mmol; formic acid, 1 ml; HfCl 4 , 0.03 mmol; DMF, 4 ml. Bulk synthesis Larger scale syntheses were also carried out to furnish sufficient material for stability studies. Standard synthetic conditions were as follows: HfCl 4 (3 mmol, 960 mg) and BDC (3 mmol, 498 mg) were added to a Schott bottle (250 ml capacity), followed by DMF (40 ml) and formic acid (95%, 20 ml). The vessel was sealed, heated to 120 °C for 24 h, then removed from the oven and allowed to cool to room temperature. The reaction mixture was subsequently filtered under vacuum and washed (acetone) to afford the required product as a white microcrystalline powder. This procedure produced the material shown in Fig. 2a . Analogous reactions in which HfCl 4 was replaced by an equimolar quantity of ZrCl 4 produced comparable results. The use of acetic acid as a modulator does not produce the nano- reo phase under these conditions, in agreement with the findings of ref. 12 . Kinetics of formation We also investigated the kinetics of formation for this system. Two reaction mixture compositions were studied: low BDC concentration, on the one hand, and high formic acid concentration, on the other hand. For the low BDC concentration series, the quantities used were as described above, except that 0.15 mmol (25 mg) BDC was used. Seven equivalent reactions were set up, with one vessel removed at every time point. For the high formic acid concentration series, the quantities used were also as described above, except that 2 ml formic acid was used. Six equivalent reactions were set up in this case, with one vessel removed at every time point. The variations in peak intensity and sharpness with time are shown in Supplementary Fig. 8 . X-ray powder diffraction measurement All samples were assessed for crystallinity and purity via their X-ray powder diffraction patterns, measured using a Philips PW1730 diffractometer (Cu K α radiation, λ =1.541 Å) over the angular (2θ) range 3–39°, using a step size of 0.02° and a scan speed of 0.02° s −1 . For quantitative analysis of peak widths and intensities, higher quality diffraction patterns were collected using a PANalytical X'Pert PRO diffractometer (Cu Kα 1 radiation, λ =1.54060 Å). Diffraction data were measured over the angular range 3–8°, with a step size of 0.002° and a scan speed of 0.006° s −1 . Diffraction patterns at elevated temperatures were collected in the angular range 3–70° using a Siemens D5000 diffractometer (Cu K α radiation, λ =1.541 Å) equipped with an Anton Paar HTK1200 furnace. Structural refinements were performed using Pawley and Rietveld strategies as implemented within the TOPAS Academic structure refinement software [33] . Extraction of quantitative peak information was not carried out within the context of a given structural model; rather, the pattern was fitted in terms of three independent peaks and a single background term. The weaker (100) and (110) reflections were modelled as Gaussians and the (111) as a split Pearson VII-type peak. In the case that a peak was clearly absent from the diffraction pattern, it was not included in the fitting process. For some samples, such as those synthesized using very high concentrations of formic acid (that is, >2.4 ml for the conditions above) and/or very low concentrations of terephthalic acid (that is, <0.1 mmol for the conditions above), additional impurity peaks appeared in the diffraction pattern. These peaks are a result of what appear to be hafnium formate phases and were included in the model wherever appropriate. These do, however, cause substantial variation in the intensity of nano- reo superlattice reflections, making interpretation of the data for these extreme cases more complex. Synthesis of these phases from reaction mixtures containing no BDC are reported in Supplementary Methods ; X-ray powder diffraction patterns are reported in Supplementary Figs 21,22 . The low-resolution structure solution of one impurity phase is reported in Supplementary Methods . Crystallographic details for the solution reported are given in Supplementary Table 4 and illustrations of this structure are given in Supplementary Figs 23, 24 . The data presented in Fig. 2f,g of the manuscript were determined from the relative intensities of the superlattice and parent reflections, the values of which are given in Supplementary Tables 5,6 . Electron microscopy In order to prepare the sample for TEM observation, the UiO-66(Hf) powder was dispersed in ethanol and the solution was sonicated for a period of 4 min. A single drop of the solution was then transferred to a copper grid coated with holey carbon and dried in air. The TEM observations were made on a JEOL JEM-2100 microscope equipped with a LaB 6 electron gun and operated at 200 kV. The TEM images and electron diffraction patterns were recorded on a Gatan ES500W side-entry CCD camera. For the nano- reo sample, in addition to the imaging and electron diffraction experiments presented in Fig. 3a,b , high-angle annular dark-field scanning transmission electron microscopy imaging ( Supplementary Fig. 1a ), energy dispersive spectroscopy ( Supplementary Fig. 2 ) and energy dispersive spectroscopy elemental mapping ( Supplementary Fig. 1b–d ) were also performed, using a JEOL JEM-2100F microscope equipped with a field-emission gun and operated at 200 kV. Due to the high susceptibility of the samples to electron beam damage, HRTEM images could not be obtained. High-angle annular dark-field scanning transmission electron microscopy images were also obtained of the fcu sample, shown in Supplementary Fig. 3 . A comparison of the electron diffraction pattern from Fig. 3a with those predicted from our models is shown in Supplementary Fig. 4 . Along with these two samples, we obtained scanning electron microscope images (Hitachi S-520) of samples synthesized with varying concentrations of formic acid (1.0–2.0 ml) ( Supplementary Fig. 25 ). Particle size appears to increase with modulator quantity, as previously noted for modulated synthesis of UiO family materials [34] . High-energy anomalous scattering Anomalous synchrotron X-ray powder diffraction measurements were performed at the I15 beamline, Diamond Light Source. A finely ground polycrystalline sample of nano- reo UiO-66(Hf) was mixed in equal mass proportions with a ceria calibration standard in a 1 mm quartz capillary and mounted in vertical geometry on the diffractometer. Angular dispersive powder diffraction data were collected using 240 s exposures first at 55 keV and then at intervals of 5 eV for a 50 eV range across the Hf K-edge (located via an I / I 0 scan using diodes placed before and after the sample) using a Perkin Elmer flat panel detector mounted 1.124 m downstream of the sample. X-ray energies were selected using a Si(111) double crystal monochromator with a divergence limited bandpass of 10 −3 . The X-ray beam was subsequently focussed to 65 μm × 65 μm and passed through a pinhole 70 μm in diameter. Diffraction patterns were measured at three different heights (offset from each other by 0.1 mm) at both 55 keV and 65.340 keV to account for any potential sample inhomogeneity. Two-dimensional powder diffraction data were calibrated using the Bragg reflections of the ceria internal standard using DAWN data analysis software (available at www.dawnsci.org ). The two-dimensional data were masked to remove contributions from dead pixels and the beamstop, and reduced to one dimensional (2θ, I ) data using PyFAI [35] . Integrated intensities were then extracted for the lowest angle peaks (the {100} and {110} reflections) by subtracting a symmetric quartic background term; the corresponding raw data are given in Supplementary Table 7 . The extracted intensities showed no evidence of systematic sample inhomogeneity. On analysis of the sample, it became clear that the sample exhibited reasonably strong beam sensitivity both at (65.34 keV) and well away (55 keV) from the edge and that the effect of radiation damage over extended exposure was an order of magnitude larger than any effect due to the anomalous scattering ( Supplementary Fig. 26 ). As a result, all analysis was carried out on diffraction patterns measured on pristine samples that had not previously been exposed to the beam; comparisons were only made between data sets that had been exposed for precisely the same amount of time. This meant that the ‘on edge’ energy we used was slightly below the actual absorption edge, because our measurements at the edge itself were only performed on regions of sample that had previously been exposed to the beam. In spite of this limitation, the predicted value of Δ f ′ between 55 keV and 25 eV below the edge is 4.7 e − ; a difference of 7%, and consequently we still expect to see a variation in diffraction intensities of up to 10% by comparing diffraction patterns collected at 55 and 65.34 keV ( Supplementary Fig. 27 ). X-ray total scattering X-ray PDF measurements were performed using powder samples of UiO-66(Hf) of varying defect concentration that were loaded in 1 mm quartz capillaries and mounted on a PANalytical Empyrean diffractometer equipped with a Mo X-ray tube ( λ =0.71 Å, Q max =17.7 Å −1 ), Mo focussing mirror and scintillation point detector. Divergence 1/4 ° , Ta), anti-scatter and Soller (0.02 rad) slits were used to adjust the incident beam profile; a programmable receiving slit, set to a height of 1 mm, was used for the diffracted beam. Total scattering data were collected over the angular range 2.75> 2θ >140°, yielding data with useable Q max =15 Å −1 . These data were corrected for background, Compton, and multiple scattering and beam attenuation by the sample container using the GudrunX package [36] , [37] . The normalized structure factor F ( Q ) was converted to the PDF in the form of the D ( r ) function as defined in ref. 38 . Experimental F ( Q ) and D ( r ) functions for both the fcu and nano- reo phases are shown in Supplementary Fig. 28a,b . In order to check that the measured PDFs were consistent with the average structure of UiO-66(Hf), we fitted the processed D ( r ) ( G ( r ) in the PDFGui formalism) using the PDFGui programme [39] . PDFGui is a ‘small-box’ refinement technique where the PDF is modelled using a crystallographic unit cell, where the lattice parameters, atom coordinates and atomic displacement parameters can be refined. As the measured PDFs do not contain information about the longer range correlations, we modelled both the defective and non-defeective UiO-66(Hf) using the non-defective average structure of ref. 13 . As hafnium has more electrons than all other atoms in the materials by an order of magnitude, it proved possible to account for nearly all the features of the experimental PDF with just the Hf–Hf and Hf–O partial correlation functions. This was done by refining the lattice parameter, the Hf position and atomic displacement parameter, the O position, an overall scale factor and a peak sharpening parameter (to allow for the differential broadening within and between clusters) defined with a cut-off of r cut =7 Å. The corresponding crystallographic details are summarized in Supplementary Tables 8,9 and the fits to data are shown in Supplementary Fig. 29c,d. Defect nanoregion model generation The defect nanoregion model was produced using a domain growth approach. For a given defect composition and cluster size, a stoichiometric 24 × 24 × 24 supercell of the fcu (ordered) UiO-66(Hf) structure was taken, and a suitable number of randomly selected Hf 6 clusters were removed. These incipient vacancy nanodomains were grown using an iterative approach as follows. First, a vacant cluster site was picked at random. Then, if it corresponded to a vacant site on the surface of a nanodomain, a neighbouring cluster site in one of the ‹100› directions was picked. If the cluster was present and not adjacent to a nanodomain of different orientation, it was removed; otherwise, it was left unchanged. This was repeated until the total vacancy concentration reached the desired value. The corresponding X-ray diffraction pattern was then calculated from the remaining atom coordinates, assuming that the contribution from any remnant guest species could be neglected and that the Hf 6 cluster coordination near defect sites was completed with formate counterions. More details of the modelling calculations are available in the Supplementary Methods and calibration curves for concentration and domain sizes are shown in Supplementary Fig. 7 . Quantum mechanical calculations The fcu and reo structures of UiO-66(Hf) were relaxed fully by optimizing both atomic positions and unit cell parameters. We performed quantum mechanical calculations in the density functional theory approach with localized basis sets (CRYSTAL09 code [40] ). We used the B3LYP hybrid exchange-correlation functional [41] and all-electron basis sets for all atoms [11] , except Hf for which we used a small relativistic effective core potential with 12 outer electrons considered explicitly [42] . The mechanical properties of both fcu and reo phases were calculated in the elastic regime, following the methodology outlined in ref. 43 . We also carried out these calculations for UiO-66(Zr) material, giving very similar results. The optimized lattice parameters, unit cell and mechanical properties are available in Supplementary Tables 1–3,10–13 . The calculation of the relative stability of the two fcu and reo phases is detailed in Supplementary Methods . Thermogravimetric analysis Samples were prepared for TGA analysis by activation under vacuum (150 °C for 24 h). TGA measurements were performed using a Perkin Elmer TGA 7, with a Perkin Elmer TAC 7/DX thermal analysis controller, from 50 to 650 °C, with a temperature ramp rate of 5 °C min −1 . The corresponding TGA traces, normalized against the mass at 650 °C, are shown in Supplementary Fig. 9 . A number of previous studies have focussed on the importance of TGA evidence for establishing ligand substoichiometry, finding ligand:cluster ratios that fall below the idealized ratio of 6:1 (ref. 44) [44] . We also find this to be the case for nanostructured UiO-66(Hf). It is also clear that with increasing modulator content the mass loss increases ( Supplementary Fig. 10 ) and hence ligand:cluster ratio decreases ( Supplementary Fig. 11 ), which is consistent with our cluster vacancy model. We also find evidence for loss of formic acid at around 250 °C, indicated by the step in mass, as previously described and seen for trifluoroacetic acid-modulated UiO-66 (ref. 20) [20] . Surface area measurements Surface area analysis was carried out by Oxford Materials Characterization Service on a systematic series of samples, prepared using varying formic acid volumes of 1.0 to 2.0 ml. All samples were activated by heating at 150 °C under dynamic vacuum for 12 h. Approximately 50 mg of activated sample was then degassed at 150 °C under a nitrogen atmosphere before BET analysis was carried out using Micromeritics Gemini V surface area analyser using nitrogen as the adsorbate. Pore diameter measurements were limited to the range 1.7–300 nm. The results of these measurements are summarized in Supplementary Table 14 . Plots illustrating the variation pore diameter, pore diameter volume and surface area, are given as Supplementary Figs 12–15 ; additional discussion regarding their interpretation is given in the Supplementary Discussion. How to cite this article : Cliffe, M. J. et al . Correlated defect nanoregions in a metal–organic framework. Nat. Commun. 5:4176 doi: 10.1038/ncomms5176 (2014).